Extensive diversification of IgH subclass-encoding genes and IgM subclass switching in crocodilians Crocodilians are a group of reptiles that are closely related to birds and are thought to possess a strong immune system. Here we report that the IgH locus in the Siamese crocodile and the Chinese alligator contains multiple μ genes, in contrast to other tetrapods. Both the μ2 and μ3 genes are expressed through class-switch recombination involving the switch region and germline transcription. Both IgM1 and IgM2 are present in the serum as polymers, which implies that IgM class switching may have significant roles in humoural immunity. The crocodilian α genes are the first IgA-encoding genes identified in reptiles, and these genes show an inverted transcriptional orientation similar to that of birds. The identification of both α and δ genes in crocodilians suggests that the IgH loci of modern living mammals, reptiles and birds share a common ancestral organization. Immunoglobulins (Igs) are essential components of the adaptive immune system and are expressed only in jawed vertebrates, including cartilaginous fish, bony fish, amphibians, reptiles, birds and mammals [1] , [2] , [3] . These defence molecules emerged ~500 million years after the divergence of jawed vertebrates from jawless vertebrates (cyclostomes such as lampreys and hagfish) [2] . No Igs are found in cyclostomes, which were recently shown to have developed a distinct recombinatorial adaptive system [4] , [5] , [6] , [7] . Antigen-binding regions (variable regions) and effector regions (constant regions) are pivotal to Ig functions. From an evolutionary perspective, comparative studies have proven to be useful in understanding how the Ig-gene variable regions have diversified and how the effector regions have multiplied (that is, the diversification of the Ig classes and subclasses) in different species [1] . A number of molecular mechanisms that are involved in shaping the IgV (V: variable) repertoire, such as V(D)J (D: diversity segments; J: joining segments) recombination, somatic hypermutation (SHM) and gene conversion, have been intensively studied. Both V(D)J recombination and SHM are utilized by all of the species that have been examined, whereas gene conversion has a major role only in birds [1] , [8] , [9] . Additionally, more than 10 genes encoding different Ig classes, such as IgM, IgD (IgW), IgNAR, IgZ (IgT), IgA (IgX), IgY, IgF, IgO, IgG and IgE, have been identified in various species [3] , [10] , [11] , [12] , [13] , [14] , [15] , [16] , [17] , [18] , [19] , [20] , and IgG and IgA are further diversified into a variable number of subclasses in mammalian species. Differential diversification of the Ig classes or subclasses may have arisen from a long evolutionary period of environmental selection pressure, thus conferring survival advantages. IgM and IgD are thought to be the most primitive Ig classes [17] , [21] , as IgM has been identified in all species examined to date and IgD is found in most species except for birds and certain mammals [22] . Logically, other IgH (H: heavy-chain genes) classes should be evolutionarily derived from IgM and IgD, likely through various mechanisms such as gene duplication, gene conversion or recombination. These processes led to the origin of IgNAR in cartilaginous fish and IgZ(T) in bony fish [13] , [14] , [23] . Although both IgY and IgA(X) appeared only after the emergence of tetrapods, the former likely preceded the latter in evolution based on the evolutionary evidence that IgA (X) resulted from a genetic recombination between IgM and IgY [24] , [25] . From lower tetrapods to mammals, IgY has been functionally diversified into IgG and IgE [26] . In addition to the insightful clues regarding Ig evolution, comparative studies have provided unexpected observations in recent decades, particularly in reptiles and birds. For example, IgD is absent in all birds examined to date [27] , although it has been identified in all other groups of jawed vertebrates, including reptiles [22] , [25] , [28] . Furthermore, although IgA (or IgX) is expressed in mammals, birds and amphibians [1] , this Ig class, which is involved in mucosal immunity, is missing in several reptiles [25] , [28] . This absence is surprising considering that even bony fish express a special Ig class, IgT, that is dedicated to mucosal immunity [15] . Notably, the α gene in birds shows a reverse transcriptional orientation to the μ and υ genes [27] . Together, these observations suggest that the IgH locus in birds and reptiles has experienced genetic rearrangements, resulting in either the deletion or inversion of certain genes. Crocodilians (including Alligatorinae, such as caimans and alligators, Crocodylinae, such as crocodiles and false gavials, and Gavialinae, such as gavials) are thought to be the closest relatives of living birds [29] . As these species provide a phylogenetic link to other reptiles and birds, analysis of their Ig genes may provide significant clues to understanding Ig evolution. Crocodilians are thought to have a strong immune system, as they are rarely subject to infection despite harsh living conditions [30] , [31] . In this study, we have therefore performed a thorough analysis of the IgH genes in two species of crocodilians: the Siamese crocodile ( Crocodylus siamensis ) and the Chinese alligator ( Alligator sinensis ). We found that the IgH locus in these species contains multiple μ genes, and that IgM subclasses can be expressed through class-switch recombination. Construction of IgH-specific mini-cDNA libraries To analyse the IgH isotypes expressed in the Siamese crocodile, we first amplified a fragment of the μ gene using degenerate primers for the conserved sequences of known μ genes in other species. We subsequently performed rapid amplification of cDNA ends (RACE) to clone the 5′-portion of IgM heavy-chain transcripts, which revealed a number of heavy-chain joining (JH) segments. It is known that in a given species of tetrapods, distinct IgH classes can share the same set of JH segments when expressed [1] . Using the JH-derived primers, we performed 3′-RACE with RNA isolated from the spleen or small intestine. The amplified 3′-RACE PCR products were cloned to construct both spleen and intestine IgH-specific mini-cDNA libraries. Theoretically, these IgH cDNA libraries should contain all of the IgH isotype transcripts provided that each transcript is expressed at a sufficient level. Multiple IgH genes are expressed in crocodilians Using PCR and sequencing, we identified 526 clones in the spleen IgH library and 428 clones in the small intestine library. Despite their different frequencies ( Supplementary Fig. S1 ), we detected heavy-chain transcripts of three distinct μ -encoding genes (termed μ1 , μ2 and μ3 , sharing 59.2 to 65% sequence identity at the protein level), three υ-encoding genes (termed υ1 , υ2 and υ3 , sharing 49.3–51.3% sequence identity at the protein level) and two α-encoding genes (termed α1 and α2 , sharing 62.4% sequence identity at the protein level) in the two libraries. A single δ heavy-chain transcript containing two CH (heavy-chain constant region) domains was also identified in the spleen library. An additional 3′-RACE reaction with primers based on the identified δ CH revealed two further transcripts: one containing four CH domains and another containing seven CH domains. The identities of these IgH genes were all confirmed by phylogenetic analysis ( Fig. 1 ). 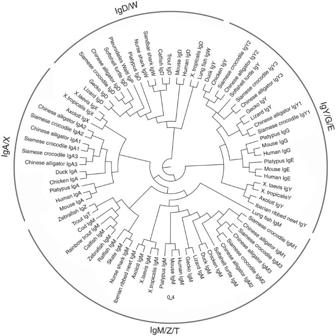Figure 1: Phylogenetic analysis of IGHC genes in jawed vertebrates. The scale bar shows the genetic distance. Figure 1: Phylogenetic analysis of IGHC genes in jawed vertebrates. The scale bar shows the genetic distance. Full size image The expression of multiple Ig subclass-encoding genes, including the μ genes, in the Siamese crocodile was unexpected because few of the tetrapod species examined thus far have been reported to express more than one μ gene. The only known exception is cattle, in which two μ genes have been detected (located in BTA21 and BTA11) [32] . To determine whether multiple Ig subclasses are expressed by other crocodilians, we analysed the IgH genes expressed in the Chinese alligator using the same approach and also detected the expression of three μ , three υ and two α heavy chains ( Supplementary Fig. S1 ). Interestingly, each of these heavy-chain transcripts corresponded with a high degree of sequence identity (>85%) to a specific class or subclass identified in the Siamese crocodile ( Supplementary Fig. S1 ), whereas the different subclasses in a single species share <70% sequence identity. These data suggest that the divergence of the Ig subclass-encoding genes likely occurred before the divergence of these two species. Physical mapping of the IgH gene locus in the Siamese crocodile We subsequently determined how these μ genes are organized in the genome, that is, whether they are organized in a single IgH locus with a ‘translocon’ structure (Vn-Dn-Jn-Cn) as in other tetrapods or in (V-D-J-Cn) clusters located on either the same or different chromosomes as found in cartilaginous fish. To address this issue, we employed genome walking to map the IgH locus of the Siamese crocodile. The corresponding genomic sequences of each IgH cDNA (except IgD) were first amplified by long-range PCR and then sequenced. These sequences served as the starting points for genome walking in both directions until overlapping sequences could be found for an upstream or downstream gene. Using this approach, we identified a genomic region of ~260 kb in which all of the identified IgH class- and subclass-encoding genes were contained. Surprisingly, an additional pseudo μ gene and two additional α genes (one structurally functional (termed α3 ) and one pseudo α ) were identified in this region ( Fig. 2a ). The pseudo μ gene was found to have a mutation at the CH1 3′-splice site (or the 5′-splice site of the following intron), changing GT AAG to AT AAG. Although the expression of the α3 gene could be confirmed at the cDNA level, the pseudo α was found to be mutated. Notably, all α genes, including the pseudo α gene, showed an opposite transcriptional orientation to all other genes within the locus. 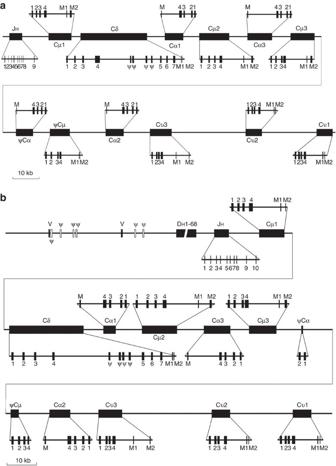Figure 2: Physical map of the IgH gene locus in two crocodilian species. (a) Physical map of the IgH gene locus in the Siamese crocodile. (b) Physical map of the IgH gene locus in the Chinese alligator. A detailed structure for each gene is also shown under or above the backbone map with the exons indicated by Arabic numerals. All of theαgenes in the locus were found to be inverted. ‘ψ’ is used to denote pseudo genes or pseudo exons. M: membrane region-encoding exon. Figure 2: Physical map of the IgH gene locus in two crocodilian species. ( a ) Physical map of the IgH gene locus in the Siamese crocodile. ( b ) Physical map of the IgH gene locus in the Chinese alligator. A detailed structure for each gene is also shown under or above the backbone map with the exons indicated by Arabic numerals. All of the α genes in the locus were found to be inverted. ‘ψ’ is used to denote pseudo genes or pseudo exons. M: membrane region-encoding exon. Full size image The δ gene was shown to have seven CH exons corresponding to the seven cloned CH-containing cDNA sequences. Additionally, four mutated CH exons were identified between δ CH4 and δ CH5 ( Fig. 2a ). It was also shown that the two cloned short IgD transcripts contained the first two and first four CH domains, respectively. The μ1 gene was located at the most 5′-end of the IGHC (Ig heavy-chain constant region gene) locus, and a JH gene locus containing nine JH gene segments was found 10 kb upstream of the μ1 gene ( Fig. 2a ). The IgH gene locus in the Siamese crocodile was arranged as JH- μ1-δ-α1-μ2-α3-μ3-ψα-ψμ-α2-υ3-υ2-υ1 . The expression of these IgH genes in different tissues was examined by quantitative RT–PCR as shown in Fig. 3 . Although all of the three μ genes were expressed at the highest levels in the spleen, both the α1 and α2 genes were expressed at the highest levels in the intestine. All three υ genes were expressed at relatively high levels in the liver and spleen. 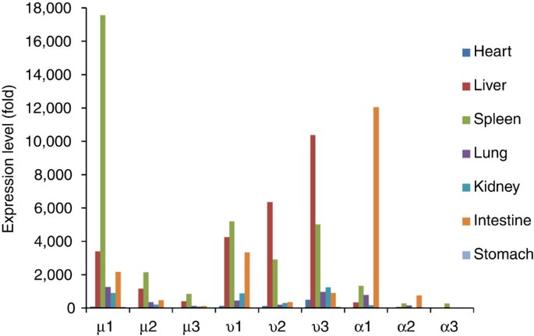Figure 3: Quantitative RT–PCR analysis of Siamese crocodile IgH gene expression in different tissues. TheEEF1A1gene was used as an internal control, and the values shown in the figure were calculated using the ΔΔCtmethod. Figure 3: Quantitative RT–PCR analysis of Siamese crocodile IgH gene expression in different tissues. The EEF1A1 gene was used as an internal control, and the values shown in the figure were calculated using the ΔΔ C t method. Full size image Physical mapping of the IgH gene locus in the Chinese alligator To analyse whether the IgH genes are similarly organized in the Chinese alligator, we generated a BAC (bacterial artificial chromosome) genomic library using peripheral blood leucocytes isolated from a Chinese alligator. The library consisted of 2.1 × 10 5 clones with an average insert size of ~100 kb ( Supplementary Fig. S2 ), representing ~9 × genomic coverage (~2.5 Gb). Five IgH gene-positive BAC clones (Y368I17, Y236C22, Y234H2, Y29J4 and Y88L23) were identified using a PCR-based approach and sequenced. Upon covering a gap between Y236C22 and Y234H2 by genome walking, we obtained a ~432 kb genomic sequence covering the alligator IgH genes. Furthermore, in addition to the genes identified at the cDNA level, a pseudo μ (ψμ), a δ , a third functional α and a pseudo α (ψα) gene were arranged in the same order as in the Siamese crocodile ( Fig. 2b ). Within nearly 200 kb upstream of the first μ, we identified two functional VH (heavy-chain variable gene), six pseudo VH, 68 DH (heavy-chain diversity segment) and 10 JH segments ( Supplementary Figs S3 and S4 ). The identification of these regions allowed us to deduce the physical map of the alligator IgH gene locus as VH n -DH (1-68) -JH (1-10) - μ1-δ-α1-μ2-α3-μ3-ψα-ψμ-α2-υ3-υ2-υ1 ( Fig. 2b ). Both the μ2 and μ3 genes are expressed through CSR In tetrapods, the expression of IgH classes other than IgM and IgD is mediated by class-switch recombination (CSR), which involves somatic DNA rearrangements that delete the μ and δ genes as well as other genes upstream of the expressed genes. As IgM is the first Ig class expressed during B-cell development, CSR switches an IgM-expressing B cell to express a non-IgM/IgD class. As two additional functional μ genes were found downstream of the most 5′ μ within the crocodilian IgH locus, we questioned whether these genes are expressed through CSR. CSR is mediated by recombination between switch (S) regions, which are located upstream of the μ gene and other IgH constant genes (except for δ ). The switch regions typically contain short, repetitive sequences that are rich in AGCT motifs. Using these criteria, we identified S regions for all of the three μ genes and υ genes in the IgH locus of the Siamese crocodile ( Supplementary Fig. S5 ). To determine whether CSR is involved in μ2 and μ3 expression, sense primers derived from the Sμ1 5′-flanking region and anti-sense primers from the Sμ2, Sμ3 and Sυ1 3′-flanking regions were designed and used in two-round nested PCR amplifications of the recombined Sμ1-Sμ2, Sμ1-Sμ3 and Sμ1-Sυ1 fragments ( Fig. 4a ). Using spleen genomic DNA as templates, these primers generated the desired bands only if somatic recombination had occurred between Sμ1 and the other S regions ( Fig. 4b ). After cloning and sequencing the amplified PCR products, we obtained 54 unique Sμ1-Sμ2 recombined fragments, 53 Sμ1-Sμ3 fragments and 45 Sμ1-Sυ1 fragments ( Fig. 4c , Supplementary Fig. S6 ), suggesting that CSR occurred between μ1 and the two downstream μ genes. 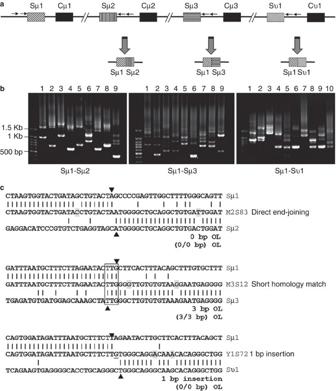Figure 4: Amplification and analysis of the recombined switch fragments Sμ1-Sμ2, Sμ1-Sμ3 and Sμ1-Sυ1. (a) Schematic demonstration of the PCR strategy used for the amplification of recombined switch fragments. (b) PCR amplification of recombined switch fragments. (c) Three representative junctions of the cloned switch fragments. For each alignment, the sequence of the cloned fragment is shown in the middle, and the germline sequences of the two S regions that are involved are shown above and below. The arrows indicate the break points, whereas boxed nucleotides denote microhomology shared by two S regions. The inserted nucleotide in the junction site is underlined. OL: overlap. Figure 4: Amplification and analysis of the recombined switch fragments Sμ1-Sμ2, Sμ1-Sμ3 and Sμ1-Sυ1. ( a ) Schematic demonstration of the PCR strategy used for the amplification of recombined switch fragments. ( b ) PCR amplification of recombined switch fragments. ( c ) Three representative junctions of the cloned switch fragments. For each alignment, the sequence of the cloned fragment is shown in the middle, and the germline sequences of the two S regions that are involved are shown above and below. The arrows indicate the break points, whereas boxed nucleotides denote microhomology shared by two S regions. The inserted nucleotide in the junction site is underlined. OL: overlap. Full size image It is well known that CSR is achieved through the non-homologous end-joining pathway in humans and mice [33] . An analysis of the junctions in the recombined fragments described above revealed a similar pattern to that observed in humans and mice [34] . Approximately one quarter (28%) of the junctions indicated direct joining of Sμ1 and the other S regions. However, more than half (57%) of the junction sites appeared to be derived from microhomology-mediated ligation, where 1–6 nucleotides were found to be shared by the two S regions involved ( Table 1 ). A small portion (16.6%) of the junctions was also shown to have nucleotide insertions between the two recombined S regions. Table 1 Summary of the junctional patterns and nucleotide mutations flanking the junction sites in the recombined switch fragments. Full size table Similar to SHM, which occurs in the variable regions of Ig genes, CSR is also an AID (activation-induced cytidine deaminase)-dependent process. In humans and mice, it has been recognized that AID can introduce mutations into S regions involved in CSR [35] . We therefore analysed the mutation pattern in the cloned switch fragments. The analysis was limited to ±25-bp sequences flanking the junction site of each recombined fragment. The analysed region accounted for 7,600 nucleotides, and a total of 120 nucleotide mutations were identified by comparison to the germline S region sequences, indicating a mutation frequency of 15.7 per 1,000 bp ( Table 1 ). Although nucleotide transitions occurred at the same rate as transversions, significantly more mutations were found at G/C sites than at A/T sites (90% versus 10%) ( Table 1 ). Approximately 73% of the mutations were located at the WRC or GYW motifs, suggesting that AID was involved in the mutational process ( Table 1 ). Identification of germline transcripts and intronic exons of μ genes In humans and mice, germline transcription through the S regions, which allows the S regions to be accessible to AID, is required to initiate CSR. Along with germline transcription, a short sequence (termed the I exon) located in the 5′ segment of each S region is spliced to the CH exons to generate germline transcripts. As μ2 and μ3 are expressed through CSR, both the I exon and the corresponding germline transcript are expected to be located upstream of these genes. Upon performing 5′-RACE to amplify the 5′- μ3 heavy-chain portion in the Siamese crocodile, we obtained three cDNAs with no rearranged VDJ sequence but with a sequence located ~0.7 kb from the 5′-Sμ3 region, which was spliced to the μ3 CH1 exon ( Fig. 5a ). This finding indicated the presence of an Iμ3 exon and germline μ3 transcription. As neither Iμ1 nor Iμ2 could be identified using the same approach, we designed a series of sense primers for the 5′-Sμ1 and -Sμ2 flanking regions. These primers were used for RT–PCR amplification together with anti-sense primers derived from μ1 and μ2 . This approach allowed us to locate Iμ1 at ~1.3 kb 5′ of Sμ1 and Iμ2 at ~0.4 kb 5′ of Sμ2 ( Fig. 5a ). Germline μ1 and μ2 gene transcripts were mainly detected in the spleen and intestine, whereas germline μ3 transcripts were mainly detected in the spleen ( Fig. 5b ). 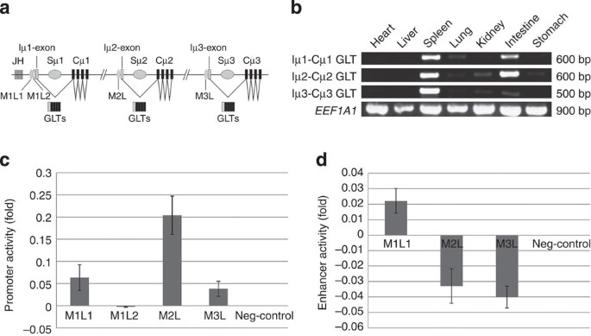Figure 5: Analysis of GL transcription, including the I promoter and enhancer for the threeμgenes. (a) Schematic map of the location of the Iμ exons and splicing of the GL transcripts. (b) GL transcription of theμgenes in various tissues. (c) Analysis of I promoter activity in the threeμgenes. (d) Analysis of enhancer activity in the three I promoters. In both (c) and (d), the pGL3-promoter or enhancer vector was used as a negative control. The Y axis indicates the relative response ratio. Data in (c) and (d) were based on three independent experiments. Error bars±s.e.m. Figure 5: Analysis of GL transcription, including the I promoter and enhancer for the three μ genes. ( a ) Schematic map of the location of the Iμ exons and splicing of the GL transcripts. ( b ) GL transcription of the μ genes in various tissues. ( c ) Analysis of I promoter activity in the three μ genes. ( d ) Analysis of enhancer activity in the three I promoters. In both ( c ) and ( d ), the pGL3-promoter or enhancer vector was used as a negative control. The Y axis indicates the relative response ratio. Data in ( c ) and ( d ) were based on three independent experiments. Error bars±s.e.m. Full size image Promoter and enhancer activity for germline transcription of μ genes Germline transcription of each Ig heavy-chain constant region gene is driven by an intronic promoter located at the 5′-region of the mammalian I exon. To determine whether there are I promoters for the Siamese crocodile μ genes, we cloned the sequences (two fragments, M1L1 and M1L2 for Iμ1, M2L for Iμ2 and M3L for Iμ3) upstream of each Iμ exon into pGL3 luciferase reporter vectors, which were then transfected into the chicken B-cell line DT40. As shown in Fig. 5c , we identified I promoters in the 5′-regions of all three Iμ exons, with M1L1, M2L and M3L fragments demonstrating promoter activities when cloned into the pGL3-enhancer vector. However, only a weak enhancer activity was detected for the Iμ1 promoter, and enhancer activity was not observed for the Iμ2 and Iμ3 promoters; only M1L1 showed enhancer activity when cloned into the pGL3-promoter vector ( Fig. 5d ), whereas M2L and M3L decreased the promoter activity to a certain extent ( Fig. 5d ). Both IgM1 and IgM2 can form polymers To examine the secreted forms of IgM in serum, we developed mouse monoclonal antibodies specific for Chinese alligator IgM1 and IgM2. Western blotting showed that under reducing conditions, both IgM1 and IgM2 heavy chains were detected as an ~80-kDa band, which is 15–20 kDa greater than the predicted size and roughly equal to the size of the mouse IgM heavy chain ( Fig. 6a ). The sizes of both IgM1 and IgM2 were reduced to approximately the predicted size when the serum sample was treated with PNGase F to remove N-linked saccharides, suggesting substantial N-linked glycosylation of both subclasses ( Fig. 6b ). The size was only slightly reduced upon O-glycosidase treatment ( Fig. 6b ). In contrast to mouse IgM (which is present as pentamers in serum), IgM1 was present as both pentamers and hexamers, whereas IgM2 was detected as tetramers under non-reducing conditions ( Fig. 6c ). 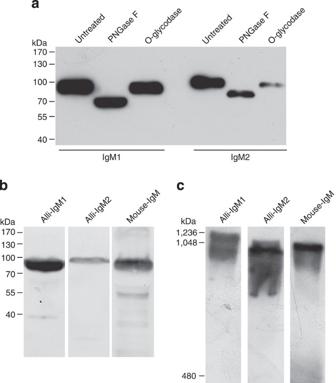Figure 6: Western blotting for IgM1 and IgM2 in the serum of a Chinese alligator. (a) Analysis of IgM1 and IgM2 treated by glycosidase under reducing conditions. (b) Analysis of IgM1 and IgM2 under reducing conditions. (c) Analysis of IgM1 and IgM2 under non-reducing conditions. In both (b) and (c), mouse serum IgM was used for comparison. Figure 6: Western blotting for IgM1 and IgM2 in the serum of a Chinese alligator. ( a ) Analysis of IgM1 and IgM2 treated by glycosidase under reducing conditions. ( b ) Analysis of IgM1 and IgM2 under reducing conditions. ( c ) Analysis of IgM1 and IgM2 under non-reducing conditions. In both ( b ) and ( c ), mouse serum IgM was used for comparison. Full size image Compared with birds and mammals, few studies have been conducted on reptilian Ig genes [25] , [28] , [36] , [37] , [38] , [39] , [40] , [41] . Crocodilians are a group of reptiles that phylogenetically link reptiles and birds, and they are thought to have a strong immune system [29] , [30] , [31] . It is thus of great interest to investigate the immunogenetic components of these crocodilians. The family Crocodylidae comprises three subfamilies (Alligatorinae, Crocodylinae and Gavialinae). The Siamese crocodile and the Chinese alligator belong to Crocodylinae and Alligatorinae, respectively. In both of these crocodilians, the IgH gene was organized similarly, as Vn-Dn-Jn- μ1-δ-α1-μ2-α3-μ3-ψα-ψμ-α2-υ3-υ2-υ1 in a ‘translocon’ configuration ( Fig. 2 ), and each IGHC gene in one species clearly had a homologous counterpart in the other species. This finding strongly suggests that Alligatorinae and Crocodylinae share a common IgH gene locus that developed before the divergence of these subfamilies ~140 million years ago [42] . This IgH gene locus is interesting in several ways. First, this locus contains orthologs of all IGHC genes found in mammals (given that the mammalian γ and ε evolved from υ ) even though the δ or α genes have not been observed in other reptiles and birds studied to date. Second, this is the first IgH gene locus in tetrapods that has been found to possess multiple μ genes. Third, it is the first IgH locus in non-mammalian tetrapods that has been shown to have subclass divergence of both the υ and α genes, although the subclass divergence of the counterparts of these genes is commonly observed in mammals. Fourth, similar to birds [27] , all of the α genes in this IgH locus showed the opposite transcriptional orientation to that of the remaining genes, indicating that α gene inversion may have occurred before the divergence of crocodilians and birds. Last, a large number (68) of DH gene segments was found in the IgH locus of the Chinese alligator, suggesting that DH segments may contribute significantly to antibody diversity in crocodilians. The present work allows us to more clearly track the evolutionary history of IgH genes in jawed vertebrates, particularly tetrapods ( Fig. 7 ). As IgM and IgD(W) are now commonly accepted to be the most primordial IgH classes in evolution [17] , [21] , [22] , it is reasonable to conclude that all other IgH classes evolved from them through various molecular mechanisms such as gene duplication, conversion or recombination. These processes gave rise to IgNAR and IgZ(T) after the divergence of cartilaginous fish and bony fish, respectively [12] , [13] , [14] . In comparison with fish, two additional IgH classes, IgY and IgA(X), have evolved in tetrapods, including amphibians, reptiles and birds. Although the origin of these classes is unknown, the present study suggests that both classes emerged before the divergence of tetrapods and that the common tetrapod ancestor expressed IgM, IgD, IgY and IgA. During tetrapod evolution, lineage-specific IgH class addition or deletion was adopted to shape the IgH locus of the modern living tetrapods. In Xenopus , the new isotype IgF, apparently derived from IgY gene duplication, was identified in addition to IgM, IgD, IgY and IgX [17] ( Fig. 7 ). Interestingly, IgA was found to be lost in a number of reptilian species, including lizards and turtles [25] , [41] , [43] , whereas IgD is absent in all birds investigated thus far [22] , [27] , [44] , [45] , [46] ( Fig. 7 ). Another important point regarding Ig evolution in tetrapods is that mammalian species inherited all IgH classes from the common tetrapod ancestor, with IgY subsequently functionally diversifying into IgG and IgE [26] . 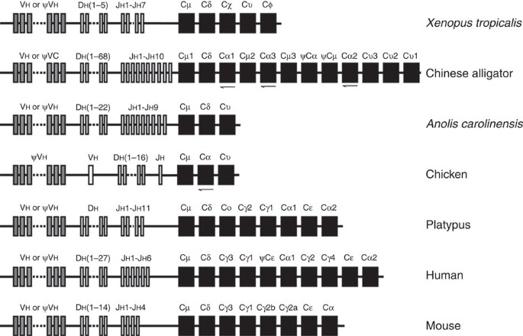Figure 7: Genomic organization of the IGHC gene locus in different species. ‘ψ’ is used to denote pseudo genes. Arrows indicate the transcriptional orientation of the chicken and Chinese alligator genes. Figure 7: Genomic organization of the IGHC gene locus in different species. ‘ψ’ is used to denote pseudo genes. Arrows indicate the transcriptional orientation of the chicken and Chinese alligator genes. Full size image The finding of three functional μ genes was unexpected. Both μ2 and μ3 genes were expressed via the CSR mechanism, which was previously shown to induce a non-IgM class switch in IgM-expressing B cells [33] . CSR is not utilized in bony or cartilaginous fish as a mechanism for expressing non-IgM/IgD antibody classes, even though the CSR initiator AID has been identified in both groups of fish [47] , [48] , [49] . Although many cis elements, such as the switch region, the I promoter and germline transcription, are required for CSR in tetrapods, none of these elements have been detected in fish [33] . Although the evolution of CSR must have been accompanied by the acquisition of these cis elements, it remains puzzling how these genetic elements were acquired by non-IgM/IgD-encoding genes. The discovery of μ to μ CSR in this study strongly suggests that these elements developed by gene duplication of the most 5′- μ gene, which is similar to the finding that multiple crocodilian μ genes likely resulted from gene duplication. Furthermore, it has long been hypothesized that non-IgM/IgD-encoding genes in tetrapods were initially derived by duplication of the μ gene [26] . In addition, as there is an Eμ enhancer with promoter activity between the JH region and the first μ in mammals and birds [33] , [50] , the I promoters of non-IgM/IgD-encoding genes are likely to be derived from the Eμ enhancer accompanying the duplication process. Identification of the crocodilian α genes in this study also provides a number of significant clues to the evolution of this gene. First, with the addition of the crocodilian α genes (representing the first bone fide reptilian α gene cloned thus far), the phylogenetic analysis clearly revealed that the α genes in reptiles, birds and mammals, as well as IgX in amphibians, share a common ancestor [51] . This finding suggests that the amphibian IgX is orthologous to IgA [51] and that the α gene emerged before the divergence of tetrapods (including amphibians, reptiles, birds and mammals). Considering the early emergence of the tetrapod α gene, it is remarkable that this antibody class, with a major importance in mucosal immunity, is missing in some reptiles [25] . Second, similar to birds, the crocodilian α genes were all inverted, suggesting that the α gene inversion also occurred before the divergence of crocodilians and birds. Third, this study provides the first evidence in non-mammalian tetrapods for the evolution of IgA subclass-encoding genes, which may have led to functional divergence and a benefit to mucosal immunity. In conclusion, this study reports the identification of a distinct IgH gene locus in crocodilians that demonstrates extensive subclass divergence of the μ , α and υ genes. Our data provide significant insight into Ig-gene evolution and improve the understanding of how a flexible Ig-gene system can develop in various species in response to long-term environmental selection pressure. Sample collection The Siamese crocodile ( Crocodylus siamensis ) was purchased from a crocodile breeding farm in Tianjin, and the Chinese alligator ( Alligator sinensis ) tissue samples were collected from the Anhui Research Centre for the Reproduction of the Chinese Alligator. Blood samples for the BAC library construction were collected from the Beijing Zoo. These studies were approved by the Animal Care and Use Committee of the China Agricultural University. BAC library construction The BAC library was constructed using a service provided by Bioestablish Biotechnology Co., Ltd (Beijing, China). Briefly, high-molecular-weight DNA was isolated from the blood cells of a Chinese alligator and embedded in agarose plugs. The DNA-containing agarose plugs were partially digested by Hin d III according to a standard protocol. The partially digested DNA was subjected to two rounds of size selection by pulsed-field gel electrophoresis in a 1% agarose gel. DNA fragments ranging from 100 to 300 kb were excised from the gel and recovered. The size-selected, digested DNA was ligated into a Hin d III-digested and dephosphorylated BAC vector. The ligation reaction was transformed into electrocompetent EPI300 cells to obtain ~2 × 10 5 recombinant clones, which were loaded onto 560 384-well plates. Super and secondary pools were also established for PCR screening. Genome walking The IgH locus of the Siamese crocodile was mapped by genome walking using a genome walking kit (Clontech, CA, USA) according to the manufacturer’s instructions. All amplifications were conducted using LA Taq DNA polymerase (Takara, Dalian, China) with proof-reading activity. Construction and screening of an IgH-specific mini-cDNA library JH-derived primers were used to perform 3′-RACE (rapid amplification of cDNA 3′-ends) using RNA isolated from the spleen and small intestine. The resultant PCR products were cloned into a pMD19-T vector. Recombinant clones were screened by sequencing and PCR. 5′-RACE amplification of the IgH heavy-chain variable regions Primers derived from the IgM heavy chain constant regions were used for 5′-RACE amplification using spleen RNA as a template. The 5′-RACE kit used was 5′-RACE System Version 2.0 (Invitrogen, NY, USA). The resultant PCR products were cloned into a pMD19-T vector and sequenced. Quantitative RT–PCR Total RNA was isolated from various tissues using an RNeasy Mini Kit (Qiagen, Valencia, CA, USA). cDNA was prepared using the QuantiTect Reverse Transcription Kit (Qiagen). The TaqMan gene expression assays were performed using the TaqMan Matrix Mix and TaqMan probes. Analysis of recombined switching fragments Two sense primers were designed using the 5′-flanking sequence of Sμ1, while six anti-sense primers (two for each S region) were designed based on the 3′-flanking sequences of Sμ2, Sμ3 and Sυ1. These primers were used for a nested PCR to amplify the recombined fragments of Sμ1-Sμ2, Sμ1-Sμ3 and Sμ1-Sυ1. The PCR was performed using the high-fidelity enzyme FastPfu DNA Polymerase (TansGen, Beijing, China). The resulting PCR products were cloned into the pMD19-T vector and sequenced. The primers sequences were as follows: M1U1 (5′-TGTGCTTGAAAGTGCATAGGA-3′) and M1U2 (5′-AACCTTGGAGCGATTTCTGAT-3′); M2L1 (5′-AACCTCTTTGAAAGCCAGCTC-3′) and M2L2 (5′-GCCACAAACCACAGAGCTAAG-3′); M3L1 (5′-ATCATCTCATTCAGCCACCTG-3′) and M3L2 (5′-TAATGGGAGAAGGCGGAAGTA-3′); and Y1L1 (5′-CACAGTGCCCAACTGGTTTAT-3′) and Y1L2 (5′-TAACCAGCCTAGCCAGTCTCA-3′). The junction sites of these recombined fragments and the mutations in the flanking regions were determined by sequence alignment with germline S regions. Promoter and enhancer activity analysis The sequences upstream of the Iμ1, Iμ2 and Iμ3 regions were cloned into both the pGL3 enhancer and pGL3-promoter vectors (Promega, WI, USA). These plasmid vectors were transfected into chicken DT40 cells using Lipofectamine 2000 (Invitrogen, NY, USA) together with the PRL-TK vector at a ratio of 1:9. The pGL3 enhancer and pGL3 control vectors were used as negative and positive controls, respectively. The activity of firefly luciferase and renilla luciferase was detected using the Dual-Glo Luciferase Assay System E2920 (Promega, WI, USA). Preparation of mAbs against the Chinese alligator IgM1 and IgM2 The mouse mAbs were prepared using a service provided by Abmart (Shanghai, China). The specificity of the obtained mAbs was confirmed by western blotting for the constant regions of IgM1 and IgM2 expressed in 293T cells. 1B2 and 3B1 mAbs were selected for the detection of IgM1 and IgM2, respectively, in the serum. Phylogenetic analysis The phylogenetic trees were constructed using MrBayes3.1.2 [52] and were viewed using FigTree or Tree View [53] . The amino-acid sequences of the entire heavy-chain constant region of most isotypes were used in the analysis, whereas the first four CH regions were used for the IgD analysis of non-mammalian vertebrates. The NCBI GenBank accession numbers of the sequences used were as follows: μ , nurse shark, M92851; skate, M29679; trout, X65261; cod, CAA41680.1; rainbow trout, AAB27359.2; zebrafish, AF281480; catfish, CAB38072.1; lung fish, AAO52808.1; Chinese soft-shelled turtle, ACU45376.1; chicken, X01613; duck, AJ314754; X. laevis , X15114; lizard, ABV66128; gecko, ABY74509; platypus, AY168639; human, X14940; mouse, V00818; X. tropicalis , AAH89670; axolotl, A46532; and Iberian ribbed newt, CAE02685; δ , catfish, U67437; X. tropicalis , DQ350886; human, BC021276; platypus, ACD31540; mouse, J00449; lizard, ABV66130; gecko, ABY67439; Chinese soft-shelled turtle, ACU45375; and trout, AAW66977; α or χ , chicken, S40610; duck, AJ314754; human, J00220; mouse, J00475; platypus, AY055778; X. laevis , BC072981; X. tropicalis , AAI57651; and axolotl, CAO82107; γ , human, J00228; mouse, J00453; and platypus, AY055781; ε , human, J00222; mouse, X01857; and platypus, AY055780; υ : chicken, X07175; duck, X78273; X. laevis , X15114; axolotl, CAA49247; lizard, ABV66132; gecko ACF60236; X. tropicalis BC089679; Chinese soft-shelled turtle, ACU45374; and Iberian ribbed newt, CAE02686; ζ / τ / π , zebrafish, AY643752; trout, AY872256; and Iberian ribbed newt, CAL25718; and ω , sandbar shark, U40560; lungfish, AF437727; and nurse shark, U51450. Statistical analysis The statistical analysis was performed using a one-way analysis of variance in SPSS1.5. Accession codes: Sequence data has been deposited in DDBJ/EMBL/GenBank under accession codes JQ417410 to JQ417429 and JQ479335 to JQ479336 . How to cite this article: Cheng, G. et al . Extensive diversification of IgH subclass-encoding genes and IgM subclass switching in crocodilians. Nat. Commun. 4:1337 doi: 10.1038/ncomms2317 (2013).